Long-life lithium-sulfur batteries with high areal capacity based on coaxial CNTs@TiN-TiO2sponge 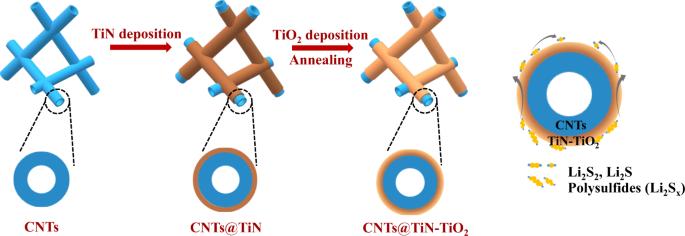Fig. 1: Schematic illustration showing the fabrication process of CNTs@TiN–TiO2and its catalytic process for the polysulfide conversion. Through the ALD method, TiN and TiO2are deposited sequentially on the CNTs surface, and then the obtained hybrid is annealed to be transformed into the coaxial CNTs@TiN-TiO2sponge with uniform distribution of the TiN–TiO2heterostructure. With the help of the TiN–TiO2heterostructure, the conversion process from lithium polysulfides to Li2S2/Li2S occurs smoothly in two steps of adsorption and catalytic conversion. Rational design of heterostructures opens up new opportunities as an ideal catalyst system for lithium polysulfides conversion in lithium-sulfur battery. However, its traditional fabrication process is complex, which makes it difficult to reasonably control the content and distribution of each component. In this work, to rationally design the heterostructure, the atomic layer deposition is utilized to hybridize the TiO 2 -TiN heterostructure with the three-dimensional carbon nanotube sponge. Through optimizing the deposited thickness of TiO 2 and TiN layers and adopting the annealing post-treatment, the derived coaxial sponge with uniform TiN-TiO 2 heterostructure exhibits the best catalytic ability. The corresponding lithium-sulfur battery shows enhanced electrochemical performance with high specific capacity of 1289 mAh g −1 at 1 C and capacity retention of 85% after 500 cycles at 2 C. Furthermore, benefiting from the highly porous structure and interconnected conductive pathways from the sponge, its areal capacity reaches up to 21.5 mAh cm −2 . Attributed to the high theoretical energy density (2600 Wh kg − 1 ), lithium–sulfur (Li–S) batteries are considered as one of the most promising candidates to meet the ever-increasing demand of high-energy rechargeable batteries [1] , [2] , [3] , [4] , [5] , [6] . However, the shuttling effect of lithium polysulfides that causes fast capacity fading and poor cycle life severely hinders practical applications of Li–S batteries [1] , [2] , [3] . To address this issue, various sulfur host materials including porous nanocarbons (e.g., graphene foam and carbon nanotube (CNT) network) and polar compounds (e.g., noncarbon oxides, sulfides, and nitrides) have been introduced to block the lithium polysulfide (Li 2 S x , 4 < x ≤ 8) shuttling physically and chemically, respectively [7] , [8] , [9] , [10] , [11] , [12] . Although these strategies can protect lithium polysulfides from being dissolved into the electrolyte to a certain extent, the shuttling problem of polysulfides is not completely solved, especially under high sulfur loadings [13] . Recent studies have shown that “dredging” other than “blocking” is a better solution to the problem of lithium polysulfide shuttling [14] . The main reason is that the conversion from lithium polysulfides to Li 2 S 2 /Li 2 S is slow during the discharging process, which will result in a large accumulation of dissolved polysulfides and eventually exceed the blocking capability of sulfur hosts. To efficiently dredge lithium polysulfides, catalysts should be introduced to accelerate the conversion rate between polysulfides and Li 2 S 2 /Li 2 S [15] , [16] . An ideal catalyst for lithium polysulfides conversion needs to be integrated with three important characteristics: (1) high electrical conductivity to promote electron and ion transport for the conversion reaction, (2) appropriate adsorption ability to stabilize polysulfides, and (3) catalytic ability to speed up the polysulfide conversion [17] . However, it is difficult to find a simple material that can simultaneously satisfy all three requirements. For example, metal oxides (such as TiO 2 ) show strong adsorption capability for polysulfides [18] , [19] , [20] , [21] , but their intrinsically low electrical conductivity will impede the polysulfides from participating in the further electrochemical reactions. Similarly, although metal nitrides (such as TiN) exhibit good electrical conductivity [22] , [23] , their weak affinities with lithium polysulfides cannot guarantee sufficient polysulfide adsorption. Recently, heterostructures that combine the advantage of each component have been introduced as improved catalysts to enhance the Li–S battery performance. For example, in the TiN–TiO 2 interlayer-based Li–S battery system, attributed to the synergistic effect of high catalytic and lithium polysulfide adsorption ability from TiN and TiO 2 , respectively, Li–S battery achieves relatively high capacity retention of 73% over 2000 cycles at 1 C [24] . The WS 2 –WO 3 heterostructure traps lithium polysulfides by WO 3 first and then transfers to WS 2 to accomplish the conversion to Li 2 S 2 /Li 2 S, realizing the capacity retention of 86.1% after 300 cycles under 0.5 C [17] . However, most of these heterostructures are synthesized by several steps including solvothermal reactions and high-temperature post-treatments. The complex fabrication process makes it difficult to reasonably control and optimize the content and distribution of each component, which play critical roles in the catalytic ability of the heterostructured catalysts. Here, we utilize the atomic layer deposition (ALD) method to fabricate a coaxial CNTs@TiN–TiO 2 sponge based on the chemical vapor deposition (CVD)-prepared three-dimensional (3D) freestanding CNT framework. Through controlling the thickness of TiO 2 and TiN layers at the outer surfaces of CNTs and combining with the annealing post-treatment, the coaxial CNTs@TiN–TiO 2 sponge derived from the CNTs hybrid with 10 nm of TiN wrapped by 5 nm of TiO 2 exhibits excellent ability to improve the Li–S battery performance with a high specific capacity of 1431 mAh g −1 at 0.2 C and high capacity retention of 85% after 500 cycles at 2 C. The main reason is that the continuous interface within the TiN–TiO 2 heterostructure makes TiO 2 adsorb lithium polysulfides first and then readily diffuses the polysulfides to TiN to proceed with the subsequent electrochemical catalysis. Meanwhile, with the synergistic contribution of highly conductive CNTs, TiN efficiently catalyzes the polysulfide conversion to Li 2 S 2 /Li 2 S. Furthermore, the porous structure and interconnected conductive pathways of the 3D CNT sponge help accommodate a large amount of sulfur and guarantee its efficient utilization. As a result, the areal capacity of the Li–S battery based on the coaxial CNTs@TiN–TiO 2 sponge reaches up to 21.5 mAh cm −2 , which is much higher than those of the commercialized lithium-ion batteries (4 mAh cm −2 ) and comparable with the recently published Li–S battery systems with the sulfur loadings higher than 8 mg cm − 2, [7] , [13] , [23] , [25] , [26] , [27] , [28] , [29] , [30] , [31] , [32] , [33] , [34] , [35] , [36] . There are three steps during the fabrication of coaxial CNTs@TiN–TiO 2 sponge: (1) depositing TiN onto CNTs following the set recipe of ALD (see the Methods for the details) to obtain CNTs@TiN, (2) growing TiO 2 layer on the outer surfaces of TiN, and (3) annealing the CNT hybrid to promote the uniform distribution of the TiN–TiO 2 heterostructure, as illustrated in Fig. 1 . The 3D porous CNT sponge is an ideal substrate for TiN–TiO 2 deposition and characterization because of the large number and special tubular structure of multi-walled CNTs, which stack layer by layer to construct the sponge. Specifically, a large number of CNTs (acting as substrates) guarantee abundant material deposition, and the deposited TiN (or TiO 2 ) can be identified readily from CNTs by transmission electron microscopy (TEM) without any complex pre-treatment in planar (or micrometer-scale) substrate-based samples, which is beneficial for the structural optimization. Moreover, numerous multi-walled CNTs within the CNT sponge interconnect with one another to provide free pathways for transporting electrons, which circumvents the electron-transport problem in thick powder-form electrodes and shows great advantage in improving the areal capacity of Li–S battery. Different from the commonly used method of loading solid sulfur as the active material, we dropped the lithium polysulfides solution to the CNTs@TiN-TiO 2 sponge, letting polysulfides soak into the sponge and act as the initial active materials directly. This is mainly for two reasons: (1) solution infiltration is one of the most feasible strategies to load active materials into 3D sulfur hosts uniformly; (2) the matched polarity between TiO 2 (or TiN) and polysulfides facilitates the efficient stabilization of active materials, which is critical for the cycling stability of Li–S battery. Benefiting from the integrated adsorption and catalytic ability of the TiN–TiO 2 heterostructure, the loaded lithium polysulfides in the CNTs@TiN–TiO 2 sponge are stabilized on the hybridized nanotubes first and then smoothly transferred to catalytic TiN to finish the conversion reaction to Li 2 S 2 /Li 2 S as shown in Fig. 1 . According to the previous report [37] , the transformation from Li 2 S 2 to Li 2 S is intrinsically a slow solid–solid reaction process, which can also be accelerated by the catalytic TiN–TiO 2 heterostructure, improving the utilization of sulfur species. Fig. 1: Schematic illustration showing the fabrication process of CNTs@TiN–TiO 2 and its catalytic process for the polysulfide conversion. Through the ALD method, TiN and TiO 2 are deposited sequentially on the CNTs surface, and then the obtained hybrid is annealed to be transformed into the coaxial CNTs@TiN-TiO 2 sponge with uniform distribution of the TiN–TiO 2 heterostructure. With the help of the TiN–TiO 2 heterostructure, the conversion process from lithium polysulfides to Li 2 S 2 /Li 2 S occurs smoothly in two steps of adsorption and catalytic conversion. Full size image Optimization of the TiN–TiO 2 heterostructure Attributed to the atomic-scale deposition and intrinsic conformity of ALD, the TiN content can be readily controlled by the deposited thickness on CNTs. Through controlling the deposition cycles, three CNT hybrids with different TiN thicknesses (5, 10, and 20 nm) are fabricated and denoted as CNTs@TiN-5, CNTs@TiN-10, and CNTs@TiN-20. From the TEM results (Fig. S1 ), the morphology of the CNTs@TiN hybrids, especially the interface between TiN and CNTs is greatly influenced by the deposited TiN thickness. Deposition of a 5 nm-thick TiN layer on the CNT surface can be clearly identified by the low magnification TEM image (Fig. S1a ), however, loose deposition on the surface of CNT with some discrete regions (Fig. S1b ) is observed under high magnification condition. As the deposited thickness of TiN increases to 10 and 20 nm, the interfaces between CNTs and TiN become continuous and smooth (Fig. S1c–f ). This morphology change is mainly attributed to the uneven surfaces of multi-walled CNTs, which impede the atomic deposition of TiN at some defective places, resulting in holes and bumps. To evaluate the electrochemical properties of these three hybrids, the Li–S cells applying them as sulfur hosts are assembled and tested. Although the battery based on CNTs@TiN-5 exhibits the highest specific capacity (about 1300 mAh g −1 ) in the first five cycles among three samples (Fig. S2 ), CNTs@TiN-10 possesses the best cycling stability with over 1000 mAh g −1 after 100 cycles, which is higher than 762 and 712 mAh g −1 of CNTs@TiN-5 and CNTs@TiN-20, respectively. By virtue of this cycling stability, it can be concluded that CNTs@TiN-10 with a continuous TiN layer is the optimized structure for the sulfur host. Although CNTs@TiN-20 has a morphology similar to that of CNTs@TiN-10, the electric conductivity measurement results show that the former has worse conductivity for electrons (Table S1 ), which substantially limits the electron transport and hinders the efficient utilization of polysulfides, resulting in lower specific capacity and inferior cyclic stability. In parallel, the loose and unstable structure of CNTs@TiN-5 is likely to be damaged during the repeated chemical reaction process, causing a fast capacity fading. Based on the above results, CNTs@TiN-10 is regarded as the optimized structure, hence it is applied as the new substrate for TiO 2 deposition. Similarly, 5 nm of TiO 2 is grown on the surface of CNTs@TiN-10 by the ALD method to fabricate the coaxial hybrid of CNTs@TiN@TiO 2 . As shown in Fig. S3a , the inner TiN can be readily distinguished from the outer TiO 2 layer of this hybrid because TiN is much coarser and looser than TiO 2 . However, the Li–S battery performance result shows that the deposited TiO 2 around the CNTs@TiN severely deteriorates the battery electrochemical performance, especially for the cyclic stability (Fig. S3b ). The dense TiO 2 layer probably blocks the diffusion of polysulfides to TiN and electron transport, which hinders the catalytic conversion of polysulfides to Li 2 S 2 /Li 2 S. In addition, the hybrids directly obtained from the ALD exhibit low crystallinity. From Fig. S4 , only one strong peak at around 26° belonging to CNTs is detected in the XRD pattern of CNTs@TiN (10 nm) and CNTs@TiO 2 (5 nm). Annealing is one of the most efficient post-treatment methods to improve the crystallinity and structures of the materials. To promote the favorable distribution of TiN and TiO 2 , CNTs@TiN@TiO 2 is annealed within dry N 2 gas atmosphere. The TEM image shows that the TiN and TiO 2 layers are mixed to form one integrated layer coated on the CNTs after annealing (Fig. 2 ) without new crystalline compound formation, which is verified by the XRD pattern of the annealed product (Fig. S5 ). The amorphous baseline in this XRD result is attributed to the amorphous carbon of the CNT sponge. The main distribution of carbon in the inner part from the corresponding EDX mapping images confirms that CNTs are applied as the original substrate for TiN and TiO 2 deposition. Interestingly, the elements of titanium, nitrogen, and oxygen wrapping around the CNTs are uniformly presented. It indicates that the annealed outer layer corresponds to a mixture of TiN and TiO 2 , which is consistent with the TEM results. From the high-resolution TEM picture (Fig. 2 ), the lattice fringes with the spacings of 0.244 and 0.324 nm are indexed to (111) lattice plane of TiN and (110) plane of TiO 2 , respectively. Besides, the TiN–TiO 2 heterostructure possesses a continuous and atomically matched interface, which is beneficial for the smooth reaction process of polysulfide adsorption, diffusion, and catalytic conversion. For the sake of concise description, the annealed CNTs@TiN@TiO 2 with TiN-TiO 2 heterostructure is named as CNTs@TiN–TiO 2 -5, of which the number stands for the thickness of the deposited TiO 2 . Because of the intrinsic conformity of the ALD method, all TiN–TiO 2 layers are uniformly grown around the outer surface of CNTs, and the hybridized CNTs@TiN–TiO 2 -5 sponge retains its porosity and 3D structure, which is beneficial for high sulfur loadings and efficient electrolyte permeation (Fig. S6 ). To further optimize the annealed TiN–TiO 2 heterostructure, two more different thicknesses of TiO 2 (2 and 10 nm) are deposited and annealed, which are denoted as CNTs@TiN–TiO 2 -2 and CNTs@TiN–TiO 2 -10. Being similar to the CNTs@TiN–TiO 2 -5, CNTs@TiN–TiO 2 -2 has an integrated TiN–TiO 2 heterostructure layer on the surface of CNTs (Fig. S6 ). 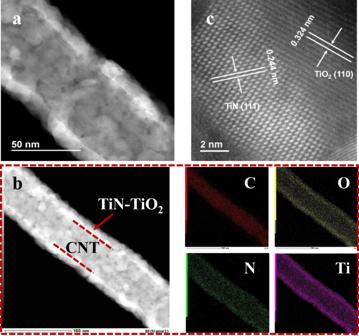Fig. 2: Morphology characterization of CNTs@TiN–TiO2-5. aTEM image of CNTs@TiN–TiO2-5 showing the integrated TiN–TiO2heterostructure coated on the CNT surface.bTEM and corresponding elemental mappings of C, O, N, and Ti in CNTs@TiN–TiO2-5 showing the mixed and uniform distribution of TiN–TiO2heterostructure.cHigh-resolution TEM of CNTs@TiN–TiO2-5 showing the well-matched interface of the TiN–TiO2heterostructure. Source data are provided as a Source Data file. However, a discontinuous and irregular boundary appears in the outer layer of the CNTs@TiN–TiO 2 -10 (Fig. S7 ). Therefore, it can be concluded that the deposited TiO 2 thickness (i.e., TiO 2 content) is an important parameter to influence the TiN–TiO 2 heterostructure. Fig. 2: Morphology characterization of CNTs@TiN–TiO 2 -5. a TEM image of CNTs@TiN–TiO 2 -5 showing the integrated TiN–TiO 2 heterostructure coated on the CNT surface. b TEM and corresponding elemental mappings of C, O, N, and Ti in CNTs@TiN–TiO 2 -5 showing the mixed and uniform distribution of TiN–TiO 2 heterostructure. c High-resolution TEM of CNTs@TiN–TiO 2 -5 showing the well-matched interface of the TiN–TiO 2 heterostructure. Source data are provided as a Source Data file. Full size image Lithium polysulfide adsorption The catalytic conversion process of lithium polysulfides includes two critical steps of the adsorption and catalytic reaction. To evaluate the adsorption ability of CNTs@TiN–TiO 2 -2, CNTs@TiN–TiO 2 -5, and CNTs@TiN–TiO 2 -10, these three hybrids are dropped into the Li 2 S 6 solution (0.005 M) and kept overnight (Fig. 3a ). The visual test result shows that the sequence of the Li 2 S 6 adsorption ability is TiO 2 > TiN > CNTs, which is consistent with the previous results. Besides, with the increase of TiO 2 content, the polysulfide adsorption ability of the CNT hybrid increases gradually. When the deposited TiO 2 thickness is 5 nm, the color of the Li 2 S 6 solution becomes transparent. However, in the Li 2 S 6 solution with CNTs@TiN–TiO 2 -2, there are still some Li 2 S 6 residues, which illustrates the limited Li 2 S 6 adsorption ability of CNTs@TiN–TiO 2 -2 and the importance of the TiO 2 content optimization (Fig. 3a ). There are two main types of adsorption between the host materials and lithium polysulfides, physical adsorption and chemical adsorption. The physical adsorption is closely correlated with the porosity (i.e., specific surface area, pore size, and pore volume) of the materials. From the BET results (Fig. S8 and Table S2 ), it can be concluded that the values of both specific surface area and mesopore volume increase with the increase of the deposited TiO 2 amount, which is beneficial for the adsorption of lithium polysulfides. However, because the strength of physical adsorption is always too weak to stabilize polysulfides efficiently, relatively strong chemical interaction in the chemical adsorption has the advantage to trap lithium polysulfides, facilitating the subsequent catalytic conversion reaction. To determine the interaction between the TiN–TiO 2 heterostructure and lithium polysulfides, X-ray photoelectron spectroscopy (XPS) measurements of CNTs@TiN–TiO 2 -5 before and after adsorption are conducted. Because of the immersion in Li 2 S 6 -contained traditional ether-based electrolyte, there is the appearance of new peaks of fluorine, sulfur, and lithium after adsorption (Fig. S9 ). As shown in Fig. 3b , the two spin–orbit splitting peaks of Ti 2 p (Ti 2 p 1/2 at 465 eV and Ti 2 p 3/2 at 459.4 eV) shift to the positions with lower binding energy (Ti 2 p 1/2 at 464.6 eV and Ti 2 p 3/2 at 458.9 eV) after Li 2 S 6 adsorption, which indicates the chemical interactions between Li 2 S 6 and TiN–TiO 2 heterostructure. Because of the stronger negativity of sulfur species than Ti, Ti 2 p tends to accept electrons from polysulfides, resulting in a lower binding energy. The formation of the new peaks of Li 3 N and N–S in N 1 s core-level region further demonstrates the chemical bonding of lithium polysulfides with the TiN–TiO 2 heterostructure (Fig. 3c ). Fig. 3: Lithium polysulfide adsorption visual test and corresponding XPS characterization of CNTs@TiN–TiO 2 -5. a Comparison of polysulfide adsorption ability of CNTs@TiN–TiO 2 -2, CNTs@TiN–TiO 2 -5, and CNTs@TiN–TiO 2 -10 by immersing these hybrids into the Li 2 S 6 solution (0.005 M). XPS spectra of b Ti 2 p and c N 1 s in CNTs@TiN–TiO 2 -5 before and after polysulfide adsorption. Source data are provided as a Source Data file. Full size image Catalytic ability A symmetric cell without the consideration of a lithium metal anode is a common configuration to evaluate the electrochemical kinetics (including the catalytic ability) of sulfur host materials. Utilizing the same material as both the cathode and anode, the symmetric cells of CNTs@TiN–TiO 2 -2, CNTs@TiN-TiO 2 -5 and CNTs@TiN–TiO 2 -10 are assembled and tested by the cyclic voltammetry (CV) method at a scanning speed of 2 mV s − 1 . Figure S10 shows that there is not any redox peak when the electrolyte without Li 2 S 6 is applied in the symmetric cells, which indicates that only Li 2 S 6 is the active material to carry out the redox reactions in the testing system, excluding the influence from the commonly used ether-based electrolyte. After Li 2 S 6 is added into the electrolyte, two pairs of redox peaks appear as shown in Fig. S10 . Specifically, two anodic peaks correspond to the oxidation of Li 2 S 2 /Li 2 S to lithium polysulfides and further to elemental sulfur (S 8 ), and two cathodic peaks are assigned to the reverse reaction process (the reduction of S 8 to polysulfides and further to Li 2 S 2 /Li 2 S). In CNTs@TiN–TiO 2 -5, these peaks exhibit narrow shapes and their separation is small, illustrating the enhanced lithium polysulfides conversion catalyzed by the TiN–TiO 2 heterostructure. In contrast, CNTs@TiN–TiO 2 -2 shows broader and wider redox peaks, suggesting the inferior catalytic capability due to the limited adsorption ability for lithium polysulfides. For CNTs@TiN–TiO 2 -10, not only the peaks are severely broadened and widened, but the current intensity is also greatly decreased, indicating the weak catalytic activity of the TiN–TiO 2 heterostructure with irregular boundaries. These unfavorable defects hinder the diffusion of the polysulfides and therefore deteriorate the catalytic ability. Besides, the inferior electric conductivity induced by the increased TiO 2 content limits the efficient utilization of lithium polysulfides. It is worth noting that Li 2 S growth is a critical step in the lithium polysulfide conversion process. To investigate the kinetics of Li 2 S precipitation (or growth), the coin cells applying Li 2 S 8 solution as the electrolyte are first galvanostatically discharged to 2.06 V and then potentiostatically discharged at 2.05 V until the current is lower than 10 −5 mA. The precipitation current and capacity can be calculated based on the potentiostat discharge curves as shown in Fig. 4 (see the Experimental section for the details). CNTs@TiN–TiO 2 -5 exhibits the highest current (0.2 mA) and capacity (328 mAh g − 1 ) for Li 2 S precipitation compared to CNTs@TiN–TiO 2 -2 (0.15 mA, 250 mAh g − 1 ) and CNTs@TiN–TiO 2 -10 (0.75 mA, 153 mAh g −1 ). These results reveal that the CNTs@TiN–TiO 2 -5 possesses the best capability to accelerate the polysulfides conversion reaction (including the Li 2 S precipitation) and promote the efficient utilization of lithium polysulfides. Fig. 4: Li 2 S deposition process under potentiostatic discharge condition. Potentiostatic discharge curves of a CNTs@TiN–TiO 2 -2, b CNTs@TiN–TiO 2 -5, and c CNTs@TiN–TiO 2 -10 at 2.05 V. Source data are provided as a Source Data file. Full size image Li–S battery performance The electrochemical measurements show that the Li–S battery applying CNTs@TiN–TiO 2 -5 as the sulfur host exhibits the best electrochemical performance including the specific capacity, rate capability, and cyclic stability. From the CV results (the scan rate is 0.1 mV s −1 ) in Fig. 5a , there are two cathodic peaks during the discharge process, corresponding to the reduction of sulfur to lithium polysulfides at higher voltage and the formation of Li 2 S 2 /Li 2 S at a lower voltage, respectively. Besides, two overlapped anodic peaks during the charging process stand for the oxidation of Li 2 S 2 /Li 2 S to lithium polysulfides and elemental sulfur. In CV curves, the separation between the corresponding cathodic and anodic peaks represents the polarization, which is correlated to the electrochemical kinetics of batteries. Theoretically, the smaller polarization reflects better electrochemical kinetics. It can be clearly observed in Fig. 5a that CNTs@TiN–TiO 2 -5 has the sharpest CV peaks, highest current intensity, and smallest polarization in comparison with CNTs@TiN–TiO 2 -2 and CNTs@TiN–TiO 2 -10. Furthermore, CNTs@TiN–TiO 2 -5 exhibits the highest discharge capacity (Fig. 5b ). In the galvanostatic charge/discharge curves, the plateaus in discharge and charge curves are attributed to the reduction and oxidation reaction processes of Li–S batteries, which agrees well with the redox peaks in CV curves (Fig. 5b ). Similarly, the gap between the discharge and charge curves also stands for the polarization, of which CNTs@TiN–TiO 2 -5 is the smallest among these three hybrids. Charge transfer resistance is an important indicator for the charge (e.g., electrons and lithium ions) transport during the battery working process. The electrochemical impedance spectroscopy (EIS) results show that CNTs@TiN–TiO 2 -5 has the smallest semicircle diameter, which corresponds to the best charge transfer capability and reveals the favorable electrochemical conversion reaction in Li–S battery with CNTs@TiN–TiO 2 -5 as the sulfur host (Fig. 5c ). For CNTs@TiN–TiO 2 -10, there are two semicircles with largely increased resistance, which illustrates that the irregular boundary in the hybrid of CNTs@TiN–TiO 2 -10 can severely limit the charge transport and the lithium polysulfide conversion reaction. Benefiting from the favorable electrochemical kinetics, CNTs@TiN-TiO 2 -5 exhibits excellent rate performance. As shown in Fig. 5d , the specific capacities of CNTs@TiN–TiO 2 -5 at the current density of 0.1, 0.5, 1, 2, and 5 C are 1350, 1250, 1000, 900, and 800 mAh g −1 , respectively. These values are much higher than that of CNTs@TiN–TiO 2 -2 and CNTs@TiN–TiO 2 -10. In addition, CNTs@TiN–TiO 2 -5 possesses the smallest polarization, and the change of the polarization value exhibits the gentlest increasing trend with the increase of the C-rate when compared to the other two hybrids of CNTs@TiN–TiO 2 -2 and CNTs@TiN–TiO 2 -10. It further verifies that the CNTs@TiN–TiO 2 -5 is an ideal host material to promote the polysulfides conversion and improve the electrochemical performance of Li–S batteries. Fig. 5: Electrochemical performance of CNTs@TiN–TiO 2 -2, CNTs@TiN–TiO 2 -5, and CNTs@TiN–TiO 2 -10. a CV curves at the scan rate of 0.1 mV s −1 , b galvanostatic charge and discharge curves, c EIS curves, and d rate performance from 0.1 to 5 C of CNTs@TiN–TiO 2 -5, CNTs@TiN–TiO 2 -2, and CNTs@TiN–TiO 2 -10. Source data are provided as a Source Data file. Full size image Furthermore, the cycling performance of the Li–S batteries is measured and compared. From Fig. 6 , the initial specific capacities of CNTs@TiN–TiO 2 -2, CNTs@TiN–TiO 2 -5 and CNTs@TiN–TiO 2 -10 at the C-rate of 0.2 C are 1271, 1431, and 1125 mAh g −1 , respectively. After 100 cycles, the capacity of 1330 mAh g − 1 is achieved for CNTs@TiN–TiO 2 -5. In contrast, only 1021 mAh g −1 for CNTs@TiN–TiO 2 -2 and 773 mAh g −1 for CNTs@TiN–TiO 2 -10 are retained. As the current density increases to 1 C and 2 C, the capacity fading rates are kept at 0.0056% and 0.031% per cycle after 220 and 500 cycles, respectively, which are competitive values for the cyclic performance of Li–S battery compared to other related works (Table S3 ) [7] , [13] , [23] , [25] , [26] , [27] , [28] , [29] , [30] , [31] , [32] , [33] , [34] , [35] , [36] . Attributed to the 3D structure, the areal sulfur loading of CNTs@TiN–TiO 2 −5 can reach up to 15 mg cm −2 . Therefore, its highest corresponding areal capacity at 0.2 C is 21.5 mAh cm − 2 , which is much higher than the related works focusing on Li–S battery with high areal capacity [25] , [38] , [39] , [40] . Even at 1 C and 2 C, the highest areal capacity of 19.3 and 12.2 mAh cm −2 can be obtained (Figs. S11 and S12 ). The initial capacity increase during the cycling is possibly due to the activation of high-loading materials under the increased C-rate condition [30] , [41] . Correspondingly, the energy density based on the whole device is about 269.05 Wh/kg at the C-rate of 0.2 C, which is comparable to the previous works calculated on the whole deive [42] , [43] . Fig. 6: Cycling performance of CNTs@TiN–TiO 2 -2, CNTs@TiN–TiO 2 -5, and CNTs@TiN–TiO 2 -10. a Cyclic stability comparison of CNTs@TiN–TiO 2 -2, CNTs@TiN–TiO 2 -5 and CNTs@TiN–TiO 2 -10 after 100 cycles at 0.2 C. b Long-term cycling performance of CNTs@TiN–TiO 2 -5 at 1 C. Source data are provided as a Source Data file. Full size image In summary, we developed a 3D coaxial CNT hybrid coated with a TiN–TiO 2 heterostructure by the ALD method combining with post-annealing. Through optimizing the deposited TiO 2 thickness, the ideal heterostructure with the continuous interface can be obtained, which facilitates the smooth process of lithium polysulfide adsorption, diffusion, and catalytic conversion. As a result, the rate performance and cyclic stability of Li–S batteries are enhanced. Furthermore, attributed to the high sulfur loading of the 3D inter-connective network, high areal capacity can be achieved simultaneously. Our strategy might be extended to the optimization of other coaxial/layer-by-layer heterostructures and promote the formation of continuous and well-matched interfaces with promising applications in energy storage and catalysis. Materials Nitric acid (HNO 3 , AR) was purchased from Wako. Tetraglyme (99.5%), sulfur (S 8 , 99.9%), and lithium disulfide (Li 2 S, 99.9%) were ordered from Sigma-Aldrich. Tetrakis(dimethylamido)titanium was bought from Japan Advanced Chemicals. All chemicals are analytical grade without further purification. Fabrication of CNTs@TiN, CNTs@TiN@TiO 2 , CNTs@TiN–TiO 2 -2, CNTs@TiN–TiO 2 -5, and CNTs@TiN–TiO 2 -10 CNT sponge was synthesized by the CVD method. The catalyst and carbon precursors are ferrocene and 1,2-dichlorobenzene, respectively. Before depositing TiN, the CNT sponge was treated with nitric acid (70% of mass ratio) at 120 °C for 12 h, which was then washed with deionized water until neutral (pH ~7). 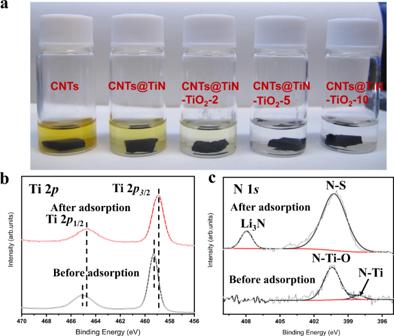Fig. 3: Lithium polysulfide adsorption visual test and corresponding XPS characterization of CNTs@TiN–TiO2-5. aComparison of polysulfide adsorption ability of CNTs@TiN–TiO2-2, CNTs@TiN–TiO2-5, and CNTs@TiN–TiO2-10 by immersing these hybrids into the Li2S6solution (0.005 M). XPS spectra ofbTi 2pandcN 1sin CNTs@TiN–TiO2-5 before and after polysulfide adsorption. Source data are provided as a Source Data file. After being freeze-dried, the CNT sponge was functionalized by carboxylic groups on the outer surfaces of CNTs, which is beneficial for the stable hybridization of sponge with other polar materials (e.g., TiN and TiO 2 ). CNTs@TiN and CNTs@TiN@TiO 2 were fabricated with the recipes at 150 °C by the ALD method in an ALD system (Cambridge Nanotechnology Savannah S200). The precursors for TiN and TiO 2 depositions are tetrakis(dimethylamido)titanium, and gases of NH 3 and H 2 O. CNTs@TiN–TiO 2 -2, CNTs@TiN–TiO 2 -5, and CNTs@TiN–TiO 2 -10 are the products of CNTs@TiN@TiO 2 being annealed in the furnace at a heating rate of 10 °C min −1 to 650 °C in flowing nitrogen (200 s.c.c.m). Recipe of CNTs@TiN (5/10/20 nm) Instruction Number Value 1 Heater 14 150 2 Heater 15 150 3 Stabilize 15 / 4 Stabilize 14 / 5 Wait / 7200 6 Pulse 4 0.15 7 Wait / 20 8 Pulse 3 0.015 9 Wait / 20 10 Goto 6 125/250/500 11 Flow / 5 Recipe of CNTs@TiN@TiO 2 (2/5/10 nm) Instruction Number Value 1 Heater 14 150 2 Heater 15 150 3 Stabilize 15 / 4 Stabilize 14 / 5 Wait / 7200 6 Pulse 4 0.15 7 Wait / 20 8 Pulse 3 0.015 9 Wait / 20 10 Goto 6 125/250/500 11 Flow / 5 12 Heater 14 150 13 Heater 15 150 14 Stabilize 15 / 15 Stabilize 14 / 16 Wait / 600 17 Pulse 4 0.5 18 Wait / 10 19 Pulse 0 0.03 20 Wait / 10 21 Goto 17 40/100/200 22 Flow / 10 Fabrication of Li 2 S 6 and symmetric cell assembly The Li 2 S 6 electrolyte was fabricated by adding Li 2 S and sulfur (molar ratio corresponds to the nominal stoichiometry of Li 2 S 6 ) into the electrolyte with 1 M lithium bis(trifluoromethane sulfonyl) imide (LiTFSI) in a mixture of 1,3-dioxolane and dimethoxyethane (1:1 in volume), and then stirring at 60 °C for 24 h. The obtained Li 2 S 6 -contained electrolyte (0.5 M) with the identical anodes and cathodes of CNTs@TiN–TiO 2 -2, CNTs@TiN–TiO 2 -5, and CNTs@TiN–TiO 2 -10 were assembled into the symmetric cells for the polysulfides conversion mechanism study. Visual test The electrodes of CNTs@TiN–TiO 2 -2, CNTs@TiN–TiO 2 -5, and CNTs@TiN–TiO 2 -10 were dropped into the diluted Li 2 S 6 electrolyte (0.005 M) and kept in the argon glove box overnight. Fabrication of Li 2 S 8 and Li 2 S precipitation test Sulfur and Li 2 S in amounts of the nominal stoichiometry of Li 2 S 8 were mixed in a tetraglyme solution at 70 °C until a dark brownish-red Li 2 S 8 solution was formed. The cells were assembled by applying CNTs@TiN–TiO 2 -2, CNTs@TiN–TiO 2 -5, and CNTs@TiN–TiO 2 -10 as the cathodes, lithium foil as anode, and Celgard 2500 membrane as the separator. 20 μL Li 2 S 8 (0.2 M) and blank electrolyte of Li–S batteries were added on the cathode and the anode, respectively. The cells were firstly discharged with a fixed current (0.134 mA) to 2.06 V to completely transform the Li 2 S 8 to Li 2 S 6 , which is followed by potentiostatically discharging at 2.05 V to convert Li 2 S 6 to Li 2 S until the current decreased to 1 × 10 −5 mA. During the potentiostatic discharge process, time-current curves were collected to analyze the conversion from Li 2 S 4 to Li 2 S. According to the potentiostatic discharge curves (Fig. 4 ), the whole discharge process was mathematically fitted into three parts representing the reduction of Li 2 S 8 and Li 2 S 6 and the precipitation of Li 2 S. The conversion capacity was calculated based on the areas of the precipitation of Li 2 S and the weight of sulfur in the Li 2 S 8 electrolyte. Material characterization The morphology and structure of the prepared samples were analyzed by SEM (Hitachi, S-3000N) and TEM (JEOL, JEM-ARM 200F). XRD measurements were performed with a Bruker D8 Discover diffractometer (Bruker AXS, Cu X-ray source). XPS analysis was performed using an X-ray photoelectron spectrometer (XPS-AXIS Ultra HAS, Kratos) with a monochromatic Al-Kα = 1486.6 eV X-ray source. Electrical conductivities of CNTs@TiN–TiO 2 -2, CNTs@TiN–TiO 2 -5, and CNTs@TiN–TiO 2 -10 were measured by a four-probe method on a Bruker Surface Profiler (Dektak XT). Nitrogen adsorption/desorption isotherms (77 K) were measured by the specific surface area/pore size distribution measurement instrument (BELSORP MINI X). Li–S battery assembly and electrochemical characterization The obtained CNTs@TiN–TiO 2 -2, CNTs@TiN–TiO 2 -5, and CNTs@TiN–TiO 2 -10 (the average areal masses are 3.7, 3.3, and 3.1 mg cm − 2 , respectively) with Li 2 S 6 electrolyte (1.2 M) were used as freestanding sulfur cathodes. 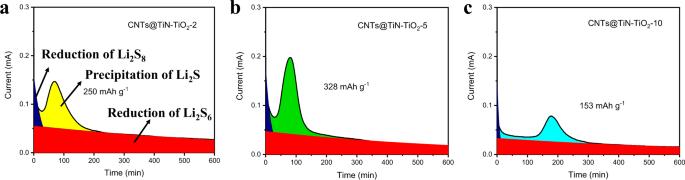Fig. 4: Li2S deposition process under potentiostatic discharge condition. Potentiostatic discharge curves ofaCNTs@TiN–TiO2-2,bCNTs@TiN–TiO2-5, andcCNTs@TiN–TiO2-10 at 2.05 V. Source data are provided as a Source Data file. 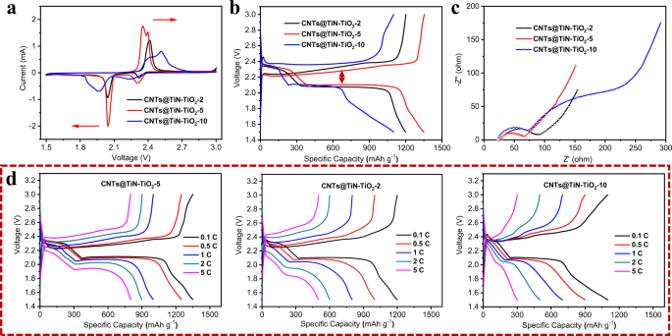Fig. 5: Electrochemical performance of CNTs@TiN–TiO2-2, CNTs@TiN–TiO2-5, and CNTs@TiN–TiO2-10. aCV curves at the scan rate of 0.1 mV s−1,bgalvanostatic charge and discharge curves,cEIS curves, anddrate performance from 0.1 to 5 C of CNTs@TiN–TiO2-5, CNTs@TiN–TiO2-2, and CNTs@TiN–TiO2-10. Source data are provided as a Source Data file. 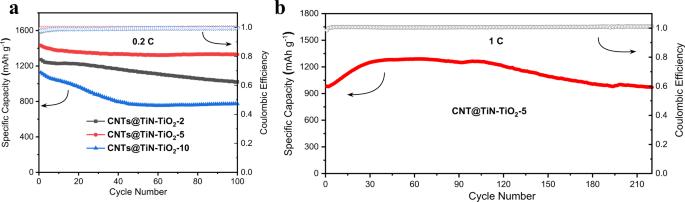Fig. 6: Cycling performance of CNTs@TiN–TiO2-2, CNTs@TiN–TiO2-5, and CNTs@TiN–TiO2-10. aCyclic stability comparison of CNTs@TiN–TiO2-2, CNTs@TiN–TiO2-5 and CNTs@TiN–TiO2-10 after 100 cycles at 0.2 C.bLong-term cycling performance of CNTs@TiN–TiO2-5 at 1 C. Source data are provided as a Source Data file. Lithium metal foils and polypropylene (PP) films (Celgard 2400) were applied as anodes and separators, respectively. The electrolyte was the 1,3-dioxolane and dimethoxyethane (1:1 volume) solution containing 1 M LiTFSI and 1 wt% lithium nitrate. Coin-type (CR 2032) cells were assembled in an argon-filled glove box. The sulfur loading and the electrolyte to sulfur mass ratio were 15 mg cm −2 and 10 µL mg − 1 , respectively. The equation of Ca = Cg × Ma was used to calculate the areal capacity of coin cells, where Ca, Cg, and Ma stand for areal capacity, specific capacity, and areal sulfur loading, respectively. The gravimetric energy density of the cell can be calculated based on the equation of E g = f × Cg × V , where f , Cg, and V stand for sulfur weight fraction of the whole device, specific capacity, and cell voltage ( V = 2.2 V), respectively. A galvanostatic electrochemical test of the assembled cells was carried out on a Neware system in the potential range of 1.5–3.0 V at different discharge/charge current densities of 0.1–5 C. CV and EIS measurements were performed on a Metrohm Autolab electrochemical workstation. EIS curves were obtained by applying a sine wave with an amplitude of 5 mV over the frequency range from 100 kHz to 0.01 Hz.